Pressure-induced chemistry in a nitrogen-hydrogen host–guest structure New topochemistry in simple molecular systems can be explored at high pressure. Here we examine the binary nitrogen/hydrogen system using Raman spectroscopy, synchrotron X-ray diffraction, synchrotron infrared microspectroscopy and visual observation. We find a eutectic-type binary phase diagram with two stable high-pressure van der Waals compounds, which we identify as (N 2 ) 6 (H 2 ) 7 and N 2 (H 2 ) 2 . The former represents a new type of van der Waals host–guest compound in which hydrogen molecules are contained within channels in a nitrogen lattice. This compound shows evidence for a gradual, pressure-induced change in bonding from van der Waals to ionic interactions near 50 GPa, forming an amorphous dinitrogen network containing ionized ammonia in a room-temperature analogue of the Haber–Bosch process. Hydrazine is recovered on decompression. The nitrogen–hydrogen system demonstrates the potential for new pressure-driven chemistry in high-pressure structures and the promise of tailoring molecular interactions for materials synthesis. The chemistry and equations of state of simple molecular systems (for example, N 2 , H 2 , H 2 O, CO 2 , CH 4 and so on) in the condensed state are of great importance to planetary astrophysics, for the accurate characterization of energetic reaction products and for engineering new molecular compounds by means of pressure-induced chemistry. These are also model systems for understanding chemical bonding, testing fundamental condensed matter theory and probing potential quantum effects at high density. Extensive studies have shown that pure N 2 and pure H 2 demonstrate subtle and complex high-pressure behaviour. In solid N 2 , quadrupole–quadrupole interactions give way to partially and later fully ordered states with increasing pressure, leading to a rich polymorphism at low-to-moderate pressures [1] . In contrast, structural changes in H 2 are determined by the interplay between quantum effects and orientational ordering, keeping the molecular centers of mass on an hcp lattice over a very large pressure domain [2] . Recent work on N 2 and H 2 has focused particular attention on the role of structure in facilitating transitions to nonmolecular and metallic phases at ultra-high pressure. A polymeric form of N 2 has been observed above 100 GPa and at high temperature, and may be an ideal high-energy density material if recoverable at ambient conditions [3] , [4] , [5] , [6] . In addition, metallic H 2 is expected to demonstrate near room-temperature superconductivity and would represent the ultimate hydride, but has thus far eluded experimental efforts [7] , [8] . Despite their fundamental nature and ubiquity, there has yet to be a comprehensive study of the full N 2 –H 2 binary system, although previous studies have examined limited individual concentrations [9] , [10] . Concentration opens a new parameter space (along with pressure and temperature) for exploring new stoichiometric compounds, reactivity in the solid solution and potential paths for the synthesis and stabilization of phases with technological applications. This could lead to new H 2 -rich compounds for fuel cell technology [11] or enable H 2 metallization by confinement in a host lattice [12] . The formation of van der Waals compounds containing N 2 and H 2 demonstrates the potential for new stoichiometries at modest pressures. The first such compounds were produced in combination with rare gases, Ar(H 2 ) 2 (ref. 13 ) and (N 2 ) 11 He (ref. 14 ). H 2 has since been shown to form a family of compounds, including (O 2 ) 3 (H 2 ) 4 (ref. 15 ), CH 4 (H 2 ) 2 (ref. 16 ), Xe(H 2 ) 7 (ref. 17 ) and SiH 4 (H 2 ) 2 (ref. 18 ). There is obvious interest in manipulating pressure-driven chemistry to transform the weak van der Waals interactions into stronger bonds, increasing the likelihood of recovering high-pressure phases at ambient conditions. Here, we examine the N 2 -H 2 binary phase diagram at 300 K to investigate both the chemistry and stability of the high-pressure solid phases. We identify two new van der Waals compounds, (N 2 ) 6 (H 2 ) 7 and N 2 (H 2 ) 2 . We study their behaviour using a combination of single-crystal X-ray diffraction in the diamond anvil cell (DAC) and Raman and infrared (IR) spectroscopy to characterize the structural, vibrational and chemical properties. (N 2 ) 6 (H 2 ) 7 presents an unexpected host–guest structure, in which an N 2 lattice hosts clusters of H 2 molecules. This compound shows evidence for a marked change from van der Waals to ionic interactions at 50 GPa and room temperature- a regime in which both end-member molecular species are otherwise quite stable. This unique pressure-induced change in bonding appears to be facilitated by the novel host–guest structure, overcoming the strong N 2 triple bond at relatively modest conditions. Binary phase diagram In this work, some 30 samples were prepared at 15 different concentrations to examine the full stoichiometric phase space as a function of pressure and to test thoroughly for reproducibility and chemical equilibrium in several regions of interest. Phase transitions were identified primarily by visual observation based on the difference in refractive index between phases, accompanied by Raman spectroscopy (described further below). We identify a eutectic-type phase diagram with at least three triple points (near 35, 60 and 80 mol% H 2 concentration) and two stoichiometric van der Waals compounds at 54 mol% and 66 mol% H 2 concentration, respectively ( Fig. 1 ). The liquidus line was determined by visual identification of the disappearance of single crystals and is represented by the locus of data points in Fig. 1a . The two species are completely miscible in the fluid phase, but have a low mutual solubility in the solid phase—<2 mol% N 2 in solid H 2 and <5 mol% H 2 in solid N 2 . The shape of the liquidus, along with visual observation, confirms the existence of two stoichiometric compounds distinguished by their disparate hexagonal and cubic symmetry ( Fig. 1b,c ). Continuous pressure measurements during decompression to the fluid state at their precise stoichiometries confirm that they melt congruently. 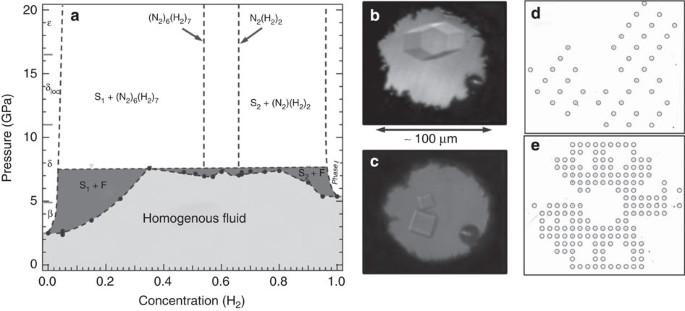Figure 1: Preliminary N2/H2binary phase diagram. (a) Fifteen concentrations were studied at room temperature. Two stoichiometric compounds exist at 54% and 66 mol% H2concentration, respectively. Away from these concentrations, phase separation occurs between the van der Waals compounds and either a nitrogen-rich solid (S1) or a hydrogen-rich solid (S2). Data points represent visual observation of complete melting. S+F indicates solid–fluid equilibrium. The (N2)6(H2)7compound has hexagonal symmetry, visual in a photomicrograph (b) of a single crystal in equilibrium with the fluid at 7 GPa. Similarly, single crystals of the N2(H2)2solid are seen to be cubic as they grow in equilibrium with the fluid, (c). Black spheres in the lower right are ruby pressure gauges. Precession images (reconstructed from the raw X-ray diffraction data) show the (h0l) layer for both solids in (d) and (e). Because of the small mosaicity of the crystals and high detector resolution, the individual points are small and therefore emphasized with circles. Figure 1: Preliminary N 2 /H 2 binary phase diagram. ( a ) Fifteen concentrations were studied at room temperature. Two stoichiometric compounds exist at 54% and 66 mol% H 2 concentration, respectively. Away from these concentrations, phase separation occurs between the van der Waals compounds and either a nitrogen-rich solid (S1) or a hydrogen-rich solid (S2). Data points represent visual observation of complete melting. S+F indicates solid–fluid equilibrium. The (N 2 ) 6 (H 2 ) 7 compound has hexagonal symmetry, visual in a photomicrograph ( b ) of a single crystal in equilibrium with the fluid at 7 GPa. Similarly, single crystals of the N 2 (H 2 ) 2 solid are seen to be cubic as they grow in equilibrium with the fluid, ( c ). Black spheres in the lower right are ruby pressure gauges. Precession images (reconstructed from the raw X-ray diffraction data) show the (h0l) layer for both solids in ( d ) and ( e ). Because of the small mosaicity of the crystals and high detector resolution, the individual points are small and therefore emphasized with circles. Full size image Structural study We identify these compounds as (N 2 ) 6 (H 2 ) 7 and N 2 (H 2 ) 2 , respectively, on the basis of their H 2 concentrations and single-crystal X-ray diffraction analyses. Samples were prepared as close to the ideal stoichiometries as possible such that the single-crystals could be grown to fill the sample chamber. In most cases, crystals were allowed to anneal for at least 24 h at room temperature and 1–2 GPa above the solidus before spectra were recorded. The single crystals are observed to have a small mosaicity in the X-ray data (0.05° in the detector plane), indicating that they are of high quality. X-ray diffraction reveals that the N 2 (H 2 ) 2 compound ( Fig. 1c ) crystallizes in a cubic structure with the most probable space groups being Pm-3m and Pm-3n . This is reminiscent of the cubic structure of the δ-phase of N 2 ( Pm-3n ) at similar pressures, but with a lattice parameter nearly twice as large ( a =12.349 Å at 9.2 GPa, compared with 6.112 Å for δ-N 2 at slightly lower pressure) [19] , [20] . A complete structural determination could not be achieved on the basis of the present data because of the rapid decrease of the reflection intensities with the diffraction angle, which we believe is due to orientational disorder of the molecules, as in δ-N 2 . Despite potential similarities with the case of Ar(H 2 ) 2 (ref. 13 ) and observations of AB 2 Laves phases in other van der Waals compounds [21] , we do not believe that the present N 2 (H 2 ) 2 compound represents a Laves phase. Indeed, there is only one cubic Laves phase with the MgCu 2 -type structure (Fd3m) and the ratio of effective molecular radii does not match the criteria for optimum packing expected for such a phase. Instead, it appears more likely that H 2 molecules either substitute in the N 2 lattice or assume interstitial positions, leading to the distension of the unit cell in a δ-N 2 -like structure. In contrast, the structure of the hexagonal solid, (N 2 ) 6 (H 2 ) 7 , differs entirely from the corresponding equilibrium structures in either N 2 or H 2 ( Fig. 2 ). It is also unlike a previously reported N 2 –D 2 structure [9] , which was not apparent in our experiments. Instead, we identify a novel host–guest compound with 36 N 2 and 42 H 2 molecules in a rhombohedral unit cell of R-3m space group. The lattice parameters for the conventional triple hexagonal cell are a = b =14.273(3) Å, and c =8.075(9) Å at 8 GPa. Full crystallographic details are given in Supplementary Table 1 . As illustrated in Fig. 2 , a cage-like lattice of N 2 molecules confines clusters of rotationally disordered H 2 molecules. Helical chains of N 2 molecules (emphasized in red, Fig. 2b ) extend along the <001> direction and confine intermediate N 2 molecules in a puckered hexagonal configuration (emphasized in green). These effectively form the ends of large, open polyhedral volumes ( Fig. 2c ), each of which hosts 15 H 2 molecules (two of which are shared with the neighbouring volumes, above and below, forming channels along the c -axis). This host–guest configuration is radically different from most van der Waals compounds, which often assume structures according to ideal hard-sphere packing configurations (for example, Ar(H 2 ) 2 , CH 4 (H 2 ) 2 , Xe(O 2 ) 2 ) [13] , [16] , [21] or share a close structural resemblance with one of the constituents (for example, (N 2 ) 11 He) (ref. 22 ). It is also notable that although N 2 molecules maintain rotational degrees of freedom in the pure phase (δ-N 2 ), here they are oriented. The presence of the guest H 2 molecules and the resulting quadrupolar interactions in the novel structure favour the formation of an ordered lattice, despite the average intermolecular distances being slightly greater than in pure N 2 . Cage-like structures, such as this, may represent an efficient means of ‘chemical compression’ by enhancing confinement of the guest molecules. Because of the potential for unique interactions in this novel host–guest structure, we set out to explore the physical and chemical behaviour of (N 2 ) 6 (H 2 ) 7 . 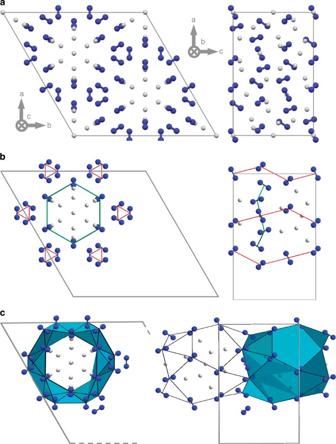Figure 2: Structure of the (N2)6(H2)7van der Waals compound. (a) Single-crystal X-ray diffraction reveals that clusters of H2molecules (shown in grey) are confined in channels within an N2lattice (blue dumbbells). (b) Helical chains of N2(emphasized in red) orient intermediate N2molecules in a puckered, hexagonal arrangement (emphasized in green) roughly in the <001> plane. (c) This generates a channel comprised of cage-like volumes along the c-axis, each of which hosts 15 H2molecules. Two of these are shared with the neighbouring volumes. Complete crystallographic data are included inSupplementary Table 1. Figure 2: Structure of the (N 2 ) 6 (H 2 ) 7 van der Waals compound. ( a ) Single-crystal X-ray diffraction reveals that clusters of H 2 molecules (shown in grey) are confined in channels within an N 2 lattice (blue dumbbells). ( b ) Helical chains of N 2 (emphasized in red) orient intermediate N 2 molecules in a puckered, hexagonal arrangement (emphasized in green) roughly in the <001> plane. ( c ) This generates a channel comprised of cage-like volumes along the c-axis, each of which hosts 15 H 2 molecules. Two of these are shared with the neighbouring volumes. Complete crystallographic data are included in Supplementary Table 1 . Full size image Raman and IR spectroscopy reveal pressure-induced chemistry Experiments were carried out on compression and decompression to 60 GPa using Raman and IR spectroscopy to investigate changes in bonding in the (N 2 ) 6 (H 2 ) 7 compound. Separate experiments were carried out to 160 GPa to track changes in IR and visible absorption. The pressure evolution of the vibron modes is shown in Fig. 3 . H 2 exhibits three IR-active vibron modes and three Raman-active modes. The highest frequency branch agrees closely in frequency and is likely shared (both Raman- and IR-active), whereas the lower frequency branches may be ascribed to different modes. All observed modes are blue-shifted with respect to pure H 2 due to partial suppression of the vibrational coupling, as observed in other H 2 /rare gas compounds [23] , [24] , [25] . In addition, the H 2 rotational mode near 600 cm −1 is seen to persist to 50 GPa, confirming that hydrogen remains rotationally free, in contrast to its N 2 host lattice ( Supplementary Fig. 5 ). Two Raman active modes and two IR active modes are observed for N 2 , with vibrational frequencies that closely follow the ν 2 mode of pure nitrogen and its branching with pressure. It is notable that IR activity begins for both species on crystallization. This is in stark contrast to the pure phases, where the IR modes appear at 20 and 215 GPa for N 2 and H 2 , respectively. This indicates an induced dipolar moment with increasing pressure, not typically present in a homonuclear diatomic molecule ( Fig. 3c ). 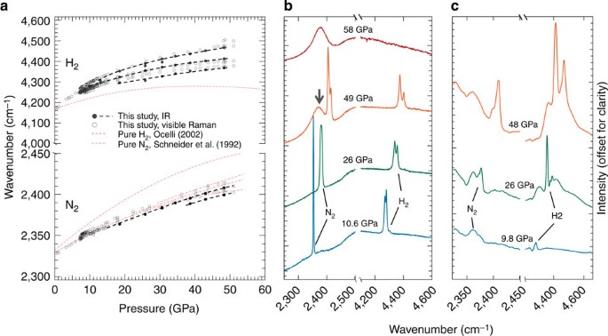Figure 3: Evidence for a chemical reaction in (N2)6(H2)7near 50 GPa. (a) Evolution of Raman and infrared vibrons for the (N2)6(H2)7inclusion compound (54 mol% H2). Red dashed curves are from refs25,45. (b) Visual Raman data taken on compression show the appearance of a new, broad feature at 2,370 cm−1, which appears near 47 GPa and grows at the expense of the υ2mode of N2with increasing pressure (indicated by an arrow). Following the appearance of this mode, the N2and H2vibrons diminish and then disappear with time (as shown at 58 GPa), suggesting a (sluggish) transition to an amorphous phase in which the previously inert molecules have reacted. (c) Infrared absorption data, also on compression, were collected on a separate sample. IR vibrons also disappear with time and with increasing pressure as a new, high-pressure phase forms from the previously crystalline solid. Figure 3: Evidence for a chemical reaction in (N 2 ) 6 (H 2 ) 7 near 50 GPa. ( a ) Evolution of Raman and infrared vibrons for the (N 2 ) 6 (H 2 ) 7 inclusion compound (54 mol% H 2 ). Red dashed curves are from refs 25 , 45 . ( b ) Visual Raman data taken on compression show the appearance of a new, broad feature at 2,370 cm −1 , which appears near 47 GPa and grows at the expense of the υ 2 mode of N 2 with increasing pressure (indicated by an arrow). Following the appearance of this mode, the N 2 and H 2 vibrons diminish and then disappear with time (as shown at 58 GPa), suggesting a (sluggish) transition to an amorphous phase in which the previously inert molecules have reacted. ( c ) Infrared absorption data, also on compression, were collected on a separate sample. IR vibrons also disappear with time and with increasing pressure as a new, high-pressure phase forms from the previously crystalline solid. Full size image At 49 GPa, a marked change in vibron signature is observed. The H 2 symmetric stretching modes disappear, whereas the N 2 Raman modes give way to a broad, lower-frequency feature ( Fig. 3b ), suggesting a possible amorphization. The amorphous state was later confirmed by the absence of X-ray diffraction peaks above the transition pressure. Despite this significant change, the solid appears to remain macroscopically intact with no visible phase separation. The transition occurs sluggishly throughout the sample, going to completion in a matter of hours and can be overdriven by as much as 15 GPa under very rapid compression. In time, however, a very broad feature appears in the Raman data in regions associated with N–H symmetric and antisymmetric stretch modes (~2,900–3,600), suggesting disruption of the strong N 2 triple bond and the onset of a chemical transformation in the amorphous, reacted solid ( Fig. 4 ). 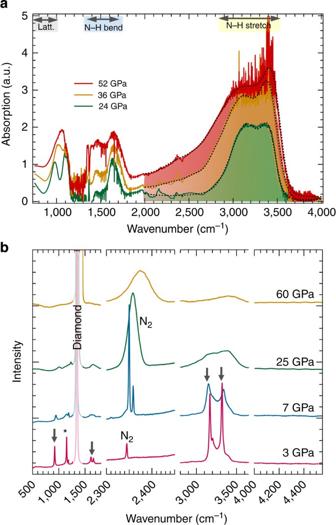Figure 4: Transition from van der Waals to ionic interactions in (N2)6(H2)7. (a) Following the pressure-induced chemical reaction in (N2)6(H2)7near 50 GPa, a broad band is observed in infrared absorption spectra above 2,000 cm−1(shaded), suggesting the presence of NH4+/NH2−in the high-pressure phase and the breakdown of van der Waals interactions in the solid. With decreasing pressure, N-H stretching modes become increasingly resolved and resemble those of NH3 (green)28, suggesting reaction of the species. (b) Visible Raman data demonstrate extreme broadening and slight redshift of the principle N2stretch mode (2,300–2,400 cm−1) in the high-pressure phase, suggesting an amorphous state. Broad N–H stretch modes (already evident at high pressure, 3,000–3,500 cm−1) become increasingly structured on decompression and are consistent with the recovery of a mixture of pure N2and hydrazine (N2H4)29,46. The peak at ~1,100 cm−1is consistent with an N–N stretch mode (indicated by a *), whereas the others (indicated by grey arrows) may be assigned to N–H bending, stretching and deformational modes. Figure 4: Transition from van der Waals to ionic interactions in (N 2 ) 6 (H 2 ) 7 . ( a ) Following the pressure-induced chemical reaction in (N 2 ) 6 (H 2 ) 7 near 50 GPa, a broad band is observed in infrared absorption spectra above 2,000 cm −1 (shaded), suggesting the presence of NH 4 + /NH 2 − in the high-pressure phase and the breakdown of van der Waals interactions in the solid. With decreasing pressure, N-H stretching modes become increasingly resolved and resemble those of NH3 (green) [28] , suggesting reaction of the species. ( b ) Visible Raman data demonstrate extreme broadening and slight redshift of the principle N 2 stretch mode (2,300–2,400 cm −1 ) in the high-pressure phase, suggesting an amorphous state. Broad N–H stretch modes (already evident at high pressure, 3,000–3,500 cm −1 ) become increasingly structured on decompression and are consistent with the recovery of a mixture of pure N 2 and hydrazine (N 2 H 4 ) [29] , [46] . The peak at ~1,100 cm −1 is consistent with an N–N stretch mode (indicated by a *), whereas the others (indicated by grey arrows) may be assigned to N–H bending, stretching and deformational modes. Full size image To better understand this transition, we probed the forward and reverse transformations in several loadings, collecting IR, Raman and visible-absorption measurements. Typical IR and Raman spectra obtained on decompression of the amorphous solid are shown in Fig. 4a,b , and suggest that the high-pressure phase has an ionic character. Most significantly, we note that IR absorption is enhanced with a broad absorption feature between ~2,100–2,900 cm −1 (shaded region, Fig. 4a ). These spectra bear a strong resemblance to recent experiments and theory on the ammonium amide phase (NH 4 + /NH 2 − ), shown to result from the auto-ionization of NH 3 , albeit at much more extreme conditions [26] , [27] , [28] . The broadband centered near 1,500 cm −1 is consistent with the bending modes of NH 4 + and NH 2 − . With increasing pressure, a strong visible absorption band is also observed between ~400–500 nm, resulting in a darkening of the sample ( Supplementary Fig. 6 ). Together with the IR data, this suggests the onset of increased charge transfer between nitrogen and hydrogen, signalling the formation of ionized NH 3 in an amorphous N 2 structure. On decompression, the visible absorption band blueshifts and decreases in intensity, accompanied by distinct structuring of N–H Raman and IR vibrational modes. The ionic character of the sample appears diminished below ~40 GPa. The breadth and relative intensity of the Raman modes are potentially consistent with an NH 3 -rich solid at higher pressures ( Fig. 4b ), however with decreasing pressure the stretching modes shift to lower frequency and become increasingly structured, evolving towards the spectral signature of N 2 H 4 hydrazine) [29] , [30] . Below 9 GPa, the N 2 vibron band progressively transforms into two well-resolved peaks close to those of pure N 2 . The solid only slightly deforms before a clear phase separation between liquid N 2 and solid N 2 H 4 , well below the melting pressure of the original (N 2 ) 6 (H 2 ) 7 compound ( Supplementary Fig. 7 ) confirming that a reaction has taken place. Excess H 2 may be present but was not detected. The structure of the (N 2 ) 6 (H 2 ) 7 compound appears to facilitate intermolecular interactions sufficient to break down the strong N≡N triple bond and promote N–H bonding above 50 GPa, resulting in chemical behaviour reminiscent of that seen in other nitrogen compounds at much more extreme conditions. Indeed, the auto-ionization of NH 3 to form ammonium amide (NH 4 + /NH 2 − ) was seen at pressures more than twice as high as our observations [27] , [28] . Mixtures of nitrogen and oxygen have also been shown to transform from molecular compounds to ionic solids (nitrosonium nitrate), though only at high temperatures [31] or when subjected to laser or X-ray irradiation [32] . Similarly, pure N 2 exhibits an amorphous, narrow band-gap, nonmolecular phase (η) but only at pressures above 150 GPa [1] , [5] , [33] , [34] , [35] . The present results demonstrate the possibility of manipulating the topochemistry of simple mixtures to markedly reduce the thresholds for pressure-induced reactions, leading to behaviour otherwise observed at much higher pressures and/or temperatures. Such high-pressure phases have tremendous potential for inducing transitions from predominantly intra- to intermolecular interactions, well within the stability regimes of the end-member constituents, as demonstrated by the observed shift from van der Waals to ionic interactions in (N 2 ) 6 (H 2 ) 7 . This is a promising avenue for exploring ‘tunable’ pressure-induced chemistry and potentially lowering activation barriers for favourable reactions in other molecular systems. We have presented a preliminary nitrogen–hydrogen binary phase diagram, which shows evidence for two new van der Waals compounds. (N 2 ) 6 (H 2 ) 7 was characterized and shown to undergo a change from van der Waals to ionic interactions coincident with a transformation to an amorphous phase near 50 GPa. On decompression, spectroscopic data show that N–H bonds evolve in the reacted solid, forming ammonium amide at high pressures and then leading to the formation of N 2 H 4 in equilibrium with liquid N 2 on melting. These results demonstrate that very interesting molecular arrangements such as the remarkable host–guest structure of (N 2 ) 6 (H 2 ) 7 can be obtained through the pressure-driven formation of van der Waals compounds. Additional stimuli (for example, photochemistry by irradiation) may further facilitate such reactions and if similar structures can be stabilized and recovered, they may represent a means of engineering solids with desirable technological applications. Other such structures may also present unique opportunities for the chemical confinement of molecular H 2 . The stability and properties of (N 2 ) 6 (H 2 ) 7 at low temperature will be the subject of future studies, and we hope that this work will motivate experimental and theoretical structural searches in other binary mixtures. Sample preparation Nitrogen–hydrogen mixtures were prepared in membrane DACs at either 20 MPa from standard bottles or 140 MPa using a gas-loading compressor. Partial gas pressures for a given concentration were calculated using a second-order virial correction to account for interaction of mixing and mixtures were left to equilibrate for at least 24 h before loading. Uncertainties in concentration are <1 mol %. Low-pressure experiments (<30 GPa) used CuBe gaskets and Boehler-Almax-type bevelled anvils with 300 μm culets. High pressures (>30 GPa) were achieved using Au-lined rhenium gaskets and diamond culets ranging from 40 to 100 μm with the sample diameter being ~1/3–1/2 that of the culet in all cases. Single crystal samples were grown under quasi-hydrostatic conditions from solid-fluid equilibrium by pressurization at room temperature and pressures were determined using the ruby fluorescence scale and/or the frequency shift of the first-order diamond phonon [36] , [37] , [38] . Spectroscopy measurements Visible Raman spectroscopy was performed in backscattering geometry and the 487.986 nm line from a continuous Ar laser, focused to ~3 μm at the sample. Data were recorded using a gain-amplified charge-coupled device (CCD) coupled to an Andor spectrometer, resulting in a spectral resolution of ~2 cm −1 . Synchrotron IR spectroscopy was carried out on the SMIS beamline at the Soleil synchrotron between 650 and 8,000 cm −1 using a coupled Fourier Transform Infrared (FTIR) spectrometer [39] . Additional IR measurements were conducted using a custom benchtop microspectroscopy system [40] . The empty DAC was used as a reference for treatment of the absorption data. X-ray diffraction and structural analysis Structural information was obtained from angle-dispersive single-crystal X-ray diffraction carried out on beamline ID09 (ref. 41 ) of the European Synchrotron Radiation Facility (Grenoble, France), using a focused (~20 μm) monochromatic beam at λ =0.4147 Å (29.8 keV). Data were recorded on a MAR 555 flat-panel detector calibrated with a Si standard. The sample was rotated in 0.5° oscillations over a range of 58° about the vertical axis during collection. CrysalisPro (Oxford Diffraction) was used to analyze the images and index reflections. The structure of the (N 2 ) 6 (H 2 ) 7 compound was solved using the ab initio charge-flipping algorithm, Superflip [42] . SHELXL [43] and Olex2 (ref. 44 ) software packages were used for structural refinement. Complete details of the structural analysis are provided in the Supplementary Discussion and Supplementary Data 1 . These techniques, together with visual microscopic observation, provide a complete suite of data on the vibrational, structural and macroscopic characteristics of the sample. How to cite this article : Spaulding, D. K. et al. Pressure-induced chemistry in a nitrogen-hydrogen host–guest structure. Nat. Commun. 5:5739 doi: 10.1038/ncomms6739 (2014).